Evolution of the base of the brain in highly encephalized human species The increase of brain size relative to body size—encephalization—is intimately linked with human evolution. However, two genetically different evolutionary lineages, Neanderthals and modern humans, have produced similarly large-brained human species. Thus, understanding human brain evolution should include research into specific cerebral reorganization, possibly reflected by brain shape changes. Here we exploit developmental integration between the brain and its underlying skeletal base to test hypotheses about brain evolution in Homo. Three-dimensional geometric morphometric analyses of endobasicranial shape reveal previously undocumented details of evolutionary changes in Homo sapiens . Larger olfactory bulbs, relatively wider orbitofrontal cortex, relatively increased and forward projecting temporal lobe poles appear unique to modern humans. Such brain reorganization, beside physical consequences for overall skull shape, might have contributed to the evolution of H. sapiens ' learning and social capacities, in which higher olfactory functions and its cognitive, neurological behavioral implications could have been hitherto underestimated factors. Accumulated palaeontological knowledge has established that the genus Homo has diversified in the last 2 million years into several evolutionary lineages, among which at least Neanderthals ( H. neanderthalensis ) and modern humans ( H. sapiens ) have independently and in parallel evolved a large brain, on average above 1400 cm 3 (refs 1 , 2 , 3 , 4 , 5 , 6 ). Clarifying the diversity in H. sapiens brain form is therefore essential for understanding cerebral evolution and functions [3] , [4] , [7] , [8] . The form of the base of the brain is well reflected in the shape of the endocranial skeletal base [9] supporting frontal lobes and olfactory bulbs within the anterior cranial fossae (ACF), and temporal lobes within the middle cranial fossae (MCF). During prenatal ontogeny the inner and outer layers of the ectomeninx, covering the developing brain, differentiate into dura mater and into precursors of the chondrocranium, which later ossifies into the endocranial base [9] , [10] . Moreover, the shape of the cribriform plate directly reflects the morphology of the olfactory bulbs, as they develop jointly [9] , [11] . 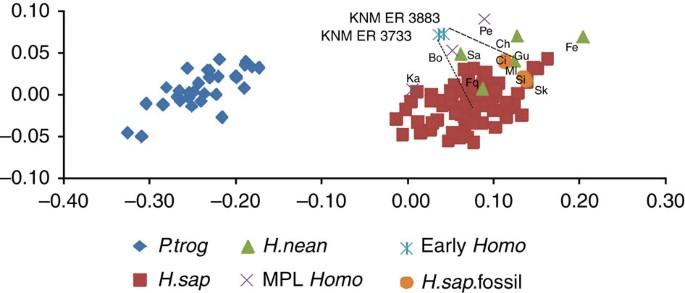Figure 1: Principal components (PC) analysis. Distributions of species along principal component (PC)1 (78.9% of total variance) and PC2 (3.4% of total variance). PC1 (abscissa) polarizes chimpanzees (negative scores) fromHomo(positive scores); PC2 (ordinate) polarizes earlyHomo(positive scores) and modern humans (negative scores). Abbreviations for fossils Ka: Broken Hill; Bo: Bodo; Pe: Petralona; Sa: Saccopastore 1; Ch: La Chapelle aux Saints; Gu: Guattari 1; Fe: La Ferrassie; Fq: Forbes' Quarry; Si: Singa; Sk: Skhul V; Ml: Mladeč 1 Ci: Cioclovina. Note divergent evolutionary patterns (indicated by arrows: dashed arrow indicating Neanderthal evolutionary lineage; dotted arrow showing modern human evolutionary lineage). Arrowheads are placed towards the centres of the Neanderthal and modern human distributions. Taking advantage of these intimate embryological and anatomical relationships, we assessed shape differences in the cranial base among large-brained humans ( Table 1 ). Specifically, we inspected the ACF to assess whether frontal widening in highly encephalized modern H. sapiens and Neanderthals differed in shape and pattern [6] , [12] . MCF were analysed to test whether modern humans evolved specifically enlarged temporal lobes [2] , [13] , [14] , [15] , [16] . These hypotheses were addressed by geometric morphometrics [17] of three-dimensional (3-D) surface landmarks of the associated endocranial cerebral base configuration ( Supplementary Fig. S1 ; Supplementary Table S1 ). Table 1 Fossil specimens. All computed tomography data except where stated STL: stereolithography). Full size table Author contributions M.B. developed the project, designed the study, collected measurements and analysed data and wrote the paper. A.R. developed the project, and worked on the manuscript. P.G. post-processed and analysed the landmark data and discussed results. A.P.M. analysed data and discussed results. G.M., K.H., R.K., C.S., J.H. provided data. All authors were involved in discussion and comments on the manuscript. Principal patterns of size and shape variation Principal components (PCs) analysis of size and shape [17] shows large-scale patterns of variation and overall distributions of data ( Fig. 1 ). PC1 distinguishes the non-human sample from Homo ( Fig. 2a,b ). PC2 polarizes early Homo versus modern humans ( Fig. 2c,d ). Large-scale shape differences show that in chimpanzees, the endocranial base of the brain is narrow, oval and elongated with a long presphenoid and a very short cribriform plate ( Fig. 2a ). In Homo ( Fig. 2b ) the base of the brain is wider and rounded, with an elongated cribriform plate and a relatively shortened pre-sphenoid. Early Homo ( Fig. 2c ) is characterized by a triangular endocranial base of the brain with a shorter cribriform plate; modern humans ( Fig. 2d ) by a rectangular base of the brain with an elongated cribriform plate. Figure 3 illustrates the mean shapes within Homo species. 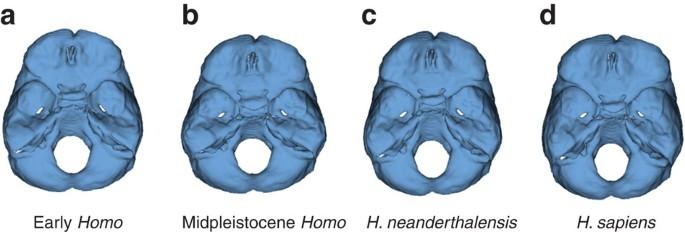Figure 3: Endocranial mean shapes. (a) EarlyHomo; (b) MidpleistoceneHomo;(c)H. neanderthalensis; (d)H. sapiens. A modern human endocranium was used to visualize the means shape by warping its endocranial surface model onto the landmark configurations of several species means. Note differences in the outlines relating to frontal and temporal lobe shapes. (a) Triangular, (b) Circular, (c) Oval, (d) Rectangular. Figure 1: Principal components (PC) analysis. Distributions of species along principal component (PC)1 (78.9% of total variance) and PC2 (3.4% of total variance). PC1 (abscissa) polarizes chimpanzees (negative scores) from Homo (positive scores); PC2 (ordinate) polarizes early Homo (positive scores) and modern humans (negative scores). Abbreviations for fossils Ka: Broken Hill; Bo: Bodo; Pe: Petralona; Sa: Saccopastore 1; Ch: La Chapelle aux Saints; Gu: Guattari 1; Fe: La Ferrassie; Fq: Forbes' Quarry; Si: Singa; Sk: Skhul V; Ml: Mladeč 1 Ci: Cioclovina. Note divergent evolutionary patterns (indicated by arrows: dashed arrow indicating Neanderthal evolutionary lineage; dotted arrow showing modern human evolutionary lineage). 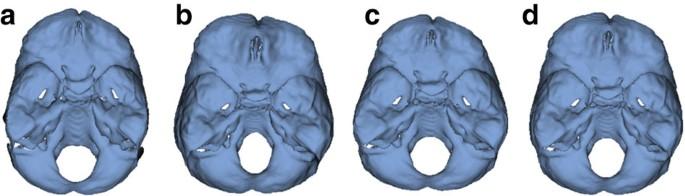Arrowheads are placed towards the centres of the Neanderthal and modern human distributions. Figure 2: Principal patterns of form variation. (a) Shape associated to negative PC1 scores; (b) shape associated to positive PC1 scores; (c) shape associated to positive PC2 scores; (d) shape associated to negative PC2 scores. Full size image Figure 2: Principal patterns of form variation. ( a ) Shape associated to negative PC1 scores; ( b ) shape associated to positive PC1 scores; ( c ) shape associated to positive PC2 scores; ( d ) shape associated to negative PC2 scores. Full size image Figure 3: Endocranial mean shapes. ( a ) Early Homo ; ( b ) Midpleistocene Homo; ( c ) H. neanderthalensis ; ( d ) H. sapiens . A modern human endocranium was used to visualize the means shape by warping its endocranial surface model onto the landmark configurations of several species means. Note differences in the outlines relating to frontal and temporal lobe shapes. ( a ) Triangular, ( b ) Circular, ( c ) Oval, ( d ) Rectangular. Full size image The covariance within the chimpanzee and hominin clouds in the PC1–PC2 plots ( Fig. 1 ) reflects the importance of size increase and allometry in brain and evolution of the base of the brain. Distributions of archaic and modern humans are roughly parallel reflecting different scaling patterns shown previously [6] . Evolutionary trajectories are indicated by lines originating close to early Homo heading towards the centres of the distribution. The Neanderthal trajectory passes in the vicinity of Petralona, a European Middle Pleistocene specimen, whereas the modern human trajectory passes through the vicinity of African Middle Pleistocene humans (Bodo, Broken Hill). For analysis of non-allometric evolutionary factors, multivariate regression analyses were performed, indicating that allometry accounts for ∼ 42% of variation ( P =0.001) in the total sample and ∼ 2.5% within Homo ( P =0.007). Non-allometric features of brain and endocranial evolution in Homo were further analysed by mean shape comparisons of the non-allometric regression residuals ( Table 2 ). Table 2 Non-allometric mean shape differences in Procrustes distance ( d ) and signifi cance levels (see also Supplementary Table S2). Full size table Statistical assessment of hypotheses Permutation tests of group membership ( N =10.000) were used to statistically assess differences in Procrustes distance [18] , [19] , [20] between non-allometric mean shapes of H. sapiens and other Homo species. Neanderthals differed significantly from the early Homo average and modern humans were highly significantly different from all other Homo species ( Table 2 ). Procrustes distance ( Table 2 ) quantifies the overall difference between means of registered landmark configurations [17] . The average distance between means within modern human populations ( d =0.037) was ∼ 25% smaller than between modern humans and Neanderthals ( d =0.049). 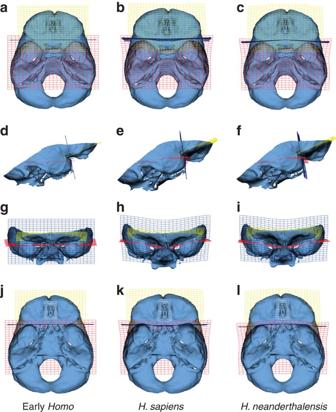Figure 4: Evolutionary transformations of mean shapes after allometry adjustment. Left column: earlyHomo; middle column:H. sapiens; right column:H. neanderthalensis. Yellow TPS grid visualizes shape change of ACF and basal frontal lobe complex; Red TPS-grid shows changes at MCF and temporal lobe complex; Dark-blue TPS-grid (vertical) delimits anterior and MCF and their associated cerebral parts. White TPS grids illustrate non-allometric evolution at the cribriform plate and olfactory bulbs. (a) Top view of undeformed earlyHomomean; (b) transformation of (a) intoH. sapiens; (c) transformation of (a) intoH. neanderthalensis. (d) Lateral view of undeformed earlyHomomean. (e) Transformation of (d) intoH. sapiens, (f) transformation of (d) intoH. neanderthalensis; (g) frontal view of undeformed earlyHomo; (h) transformation of (g) intoH. sapiens; (i) transformation of (g) intoH. neanderthalensis. (j) Inferior view of undeformed earlyHomomean. (k) Transformation of (j) intoH. sapiens. (l) Transformation of (j) intoH. neanderthalensis; note different TPS transformations pattern in earlyHomo-H. sapiensand earlyHomo -H.neanderthalensiscomparisons. (Shape difference vectors are ×1.5 magnified). However, biological understanding of these quantitative results required detailed analysis of the corresponding visualizations of the involved anatomical structures presented in Figure 4 . Figure 4: Evolutionary transformations of mean shapes after allometry adjustment. Left column: early Homo ; middle column: H. sapiens ; right column: H. neanderthalensis . Yellow TPS grid visualizes shape change of ACF and basal frontal lobe complex; Red TPS-grid shows changes at MCF and temporal lobe complex; Dark-blue TPS-grid (vertical) delimits anterior and MCF and their associated cerebral parts. White TPS grids illustrate non-allometric evolution at the cribriform plate and olfactory bulbs. ( a ) Top view of undeformed early Homo mean; ( b ) transformation of ( a ) into H. sapiens ; ( c ) transformation of ( a ) into H. neanderthalensis . ( d ) Lateral view of undeformed early Homo mean. ( e ) Transformation of ( d ) into H. sapiens , ( f ) transformation of ( d ) into H. neanderthalensis ; ( g ) frontal view of undeformed early Homo ; ( h ) transformation of ( g ) into H. sapiens ; ( i ) transformation of ( g ) into H. neanderthalensis . ( j ) Inferior view of undeformed early Homo mean. ( k ) Transformation of ( j ) into H. sapiens . ( l ) Transformation of ( j ) into H. neanderthalensis ; note different TPS transformations pattern in early Homo-H. sapiens and early Homo -H.neanderthalensis comparisons. (Shape difference vectors are ×1.5 magnified). Full size image Frontal lobes and olfactory bulbs differ in large-brained humans To investigate the evolution of the ACF, and the morphology of the associated basal part of the frontal lobes [12] we calculated thin-plates spline transformation grids (TPS-grids) [17] between the non-allometric species averages. A yellow TPS-grid passes through the limit between anterior and MCF and the anterior- and superior-most landmarks of the orbital roofs (Methods). Modern humans evolved a unique endocranial configuration at the basal frontal lobes. When compared with early Homo ( Fig. 4a ), the ACF-grid is strongly expanded mediolaterally ( Fig. 4b ). Frontal lobe widening, known for higher encephalized humans [6] , [12] , produces a rectangular outline of the frontal lobe base in H. sapiens . Maximum breadth of the basal frontal lobes is located close to the anterior half of the ACF ( Figs 3 , 4b ) at the level of the cribriform plate. At the same time the cribriform plate in the centre of the ACF, is relocated by posterior expansion. It is thus relatively larger than in early Homo and shifts the central midline base relatively backwards. The backward-flexed vertical TPS-grid ( Fig. 4b ) and the expanded white TPS-grid ( Fig. 4k ) shows this clearly ( Supplementary Movie 1 ). Neanderthals are also expanded mediolaterally but differently when compared with H. sapiens. The greatest width of the base of the frontal lobes was at the posterior half of the ACF, posterior to the cribriform plate. Further, the cribriform plate (and olfactory bulbs) was slightly increased anteriorly leading to a more oval ACF outline ( Fig. 4c,l ; Supplementary Movie 2 ). (These different evolutionary patterns were also found comparing Mid-Pleistocene fossils with modern humans and Neanderthals, Supplementary Fig. S2. ) 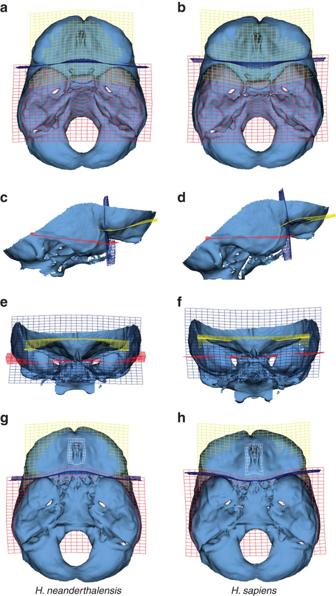Figure 5: Non-allometric differences between modern humans and Neanderthals. Shown asH. sapiens- Neanderthal (left column) and Neanderthal -H. sapiens(right column) transformations (both ×1.5 magnified). From uppermost to lowest row: superior, lateral, frontal and inferior views are shown. (a), (c), (e), and (g) Neanderthals; (b), (d), (f) and (h)H. sapiens. Note that differences are mainly recognizable in the top (a,b), lateral (c,d) and inferior (g,h) views showing lateral expansion at the ACF at the antero–lateral prefrontal cortex, significantly stronger vertical and lateral increase and forwards projection of the MCF-temporal lobe poles and enlarged cribriform plate and olfactory bulb (TPS-grid in white) in modern humans, causing a backwards retraction of the pre-sphenoid andsella turcica(gcompared withh). The significantly different evolutionary patterns in the modern human and Neanderthal lineages are shown in Figure 5 . In H. sapiens cribriform expansion has occurred posteriorly. This leads to an endocranial retraction of midline base structures relative to the lateral ACF, which projects forwards more and is relatively wider anteriorly ( Supplementary Movies 3 and 4 ). In Neanderthals, cribriform expansion is weaker and occurs anteriorly. The lateral ACF is retracted relative to the midline, which is rather stable. Figure 5: Non-allometric differences between modern humans and Neanderthals. Shown as H. sapiens - Neanderthal (left column) and Neanderthal - H. sapiens (right column) transformations (both ×1.5 magnified). From uppermost to lowest row: superior, lateral, frontal and inferior views are shown. ( a ), ( c ), ( e ), and ( g ) Neanderthals; ( b ), ( d ), ( f ) and ( h ) H. sapiens . Note that differences are mainly recognizable in the top ( a,b ), lateral ( c,d ) and inferior ( g,h ) views showing lateral expansion at the ACF at the antero–lateral prefrontal cortex, significantly stronger vertical and lateral increase and forwards projection of the MCF-temporal lobe poles and enlarged cribriform plate and olfactory bulb (TPS-grid in white) in modern humans, causing a backwards retraction of the pre-sphenoid and sella turcica ( g compared with h ). Full size image Cribriform plate enlargement in H. sapiens was further assessed comparing the lengths of the cribriform plate of three Neanderthals (Forbes Quarry: 17 mm; Saccopastore 1: 17.5 mm; Guattari 1: 23.3 mm; average: 19.16 mm) with H. sapiens (average: 22.32 mm). Owing to the small sample size of Neanderthals, non-parametric statistics were used to test the null hypothesis that cribriform length measurements from Neanderthal and modern humans were drawn from the same population. Significant differences at a P =0.0019 level ( z -adjusted P =0.025) suggested larger cribriform plates and olfactory bulbs in modern humans. Shape differences in the basal frontal lobes can either relate to the larger cribriform plate due to integration, or may imply increased neuroglia, known in primate encephalization [18] , [19] , increased gyrification [20] or increased numbers of mini columns [21] . Number and width of these, and the space between them available for interconnectivity have been discussed in the context of 'higher' cognitive functions related to prefrontal cortex [21] , among other features [22] , [23] , [24] , [25] . More importantly, arrangement of mini columns distinguishes H. sapiens from great apes [21] , in contrast to relative frontal lobe volume, which does not differ among hominoids [14] , [15] , [21] . However, evolutionary shape changes at the base of the frontal lobes shown in Figure 4 support the hypothesis of a frontal widening in higher encephalized members of Homo [12] . Nevertheless, our surface analysis reveals local differences of widening, adding spatial detail to recent allometric frontal lobe comparisons [12] . Modern human temporal lobes have an apomorphic location and size Temporal lobe morphology was approximated by quantification of 3-D endocranial surface shape of the MCF [9] , [10] , [16] . To visualize the results of quantitative non-allometric mean shape comparisons a red TPS-grid was positioned through the forward-most projection of the MCF poles, which correspond to the poles of the temporal lobes [16] . The posterior position of the TPS-grid was defined by landmarks at the base of the petrosal pyramids [26] . Transformations of the MCF–TPS-grid ( Fig. 4a,d,j into Fig. 4b,e,k ) visualize main patterns of MCF-temporal lobe evolution in modern humans. These evolutionary changes include a strong increase in relative length, seen as antero–posterior expansion of the MCF grid ( Fig. 4b ). Modern human temporal lobes are anteriorly also relatively wider (although both large-brained humans show increase in MCF width). Increased relative width of the anterior-most poles of the temporal lobes has been hypothesized [2] , [27] . Our data quantify the entire configuration of the temporal lobe poles and show that temporal lobe increase in width in modern humans has not only occurred medially to the anterior-most poles but also superolaterally ( Fig. 4b ; Supplementary Movie 1 ). Elevation of the red MCF grid in modern humans ( Fig. 4e ) suggests relative increase in height. As a result, relatively longer, wider and higher modern human temporal poles project forwards relative to the midline [16] , shown by the antero–lateral expansion of the vertical TPS-grid ( Fig. 4b ), but more clearly by bilateral forwards deformations of the vertical TPS-grid in front of the temporal lobe poles ( Fig. 4k ). The retracted area of the vertical grid in the midline is due to posterior cribriform expansion ( Fig. 4k ; Supplementary Movie 1 ). In contrast to modern humans, Neanderthal temporal lobe shape evolution does not comprise a relative elongation and forwards deformations of the vertical TPS-grid ( Fig. 4c,l ). There is increase in relative width but MCF poles remain vertically low, similar to the primitive condition ( Fig. 4d,f ; for example, early Homo ; Supplementary Movie 2 ). Retention of low temporal pole position and relative length could be seen as structural elements of Bruner et al . 's [6] hypothesis of an archaic pattern of Neanderthal encephalization. Net effects of these distinct evolutionary patterns are shown in Figure 5 ( Supplementary Movie 3 and 4 ). TPS-grid transformations of H. sapiens into Neanderthals ( Fig. 5a,c,e,g ) and Neanderthals into H. sapiens ( Fig. 5b,d,f,h ) show that modern humans still have significantly forward-projecting temporal lobe poles, that are also shifted more laterally and are still vertically increased ( Fig. 5c,d ). Inferior views demonstrate well decreased lateral width and projection in Neanderthals ( Fig. 5g ) compared with H. sapiens ( Fig. 5h ). Strong retraction of the midline base (sphenoid) due to posterior cribriform enlargement in the transformation of the Neanderthal into the modern human mean ( Fig. 5h ) leads—when transforming modern humans into Neanderthals—to a comparably strong forwards shift of the central cranial base in the latter ( Fig. 5g ). Our results confirm quantitatively previous speculations based on partial measurements on temporal lobe evolution in Homo [2] , [13] , [16] , [27] , [28] . Importantly, the mid-sagittal part of the modern human endocranium is in a more posterior position ( Fig. 5g,h ). As mentioned previously, differential expansion of the cribriform plate and olfactory bulbs appears implicated in this evolutionary change. Figure 4 suggests that non-allometric increase of the cribriform length and of the widths of the frontal lobes and temporal lobe poles are apomorphies in the large-brained human clade ( H. sapiens , H. neanderthalensis ). In a frontal view, large-brained humans also share a lower midline base relative to the lateral one ( Fig. 4g, h, and i ). H. sapiens is autapomorphic by a posteriorly enlarged cribriform plate, which shifts the central base posteriorly and roughly intersects with the maximal ACF diameter, and a forward-projection of relatively anterior and superolaterally increased temporal lobe pole relative to the central base (optic foramina; Fig. 4b,e,k ). Neanderthal autapomorphies include a cribriform plate, which is also enlarged, but anteriorly and less so than in H. sapiens , and shifted slightly anteriorly. Maximum ACF diameter passes posteriorly to the cribriform plate ( Fig. 4c,j,l ). Empirical evidence has repeatedly demonstrated that a major part of primate brain evolution is explained by brain size increase [19] , [25] , [29] . Our PCs ( Fig. 1 ) and multivariate regression analyses of shape variation at the endocranial base of the brain likely reflect this allometric factor. Nevertheless, non-allometric features have also been identified ( Table 2 , Fig. 4 ) that are suggestive of more specific interpretations [19] , [25] . Evolution in Homo is organized around modifications of the base of the brain morphology and supposedly associated functions. At a functional level of interpretation, it is clear that not all behaviourally relevant evolutionary modifications in brain connectivity and structure will be recorded in shape changes of the brain and endocranium. Our study reveals significant evolutionary modifications of the absolute and relative size of the cribriform plate, accompanied by changing configurations of the endocranial base of the temporal lobe poles and basal frontal lobes. However, evolutionary shape change of the endocranium could also reflect effects of craniofacial integration and, thus, non-cerebral factors [2] , [27] , [30] . Therefore, palaeoneurological interpretations of endocranial morphology must consider this wider spectrum of evolutionary and developmental interactions. Cribriform plate increase is well observed comparing mean shapes of modern humans with its putative ancestors (both early Homo in Figure 4 , and Mid-Pleistocene humans in Supplementary Fig. S2 ) but also with Neanderthals ( Fig. 5 ). The size of the cribriform plate is driven by the size of the olfactory bulbs due to coordinated embryological development [9] , [11] . Adult morphology of the cribriform plate is achieved early in ontogeny (4 years in humans [9] and probably even earlier in Neanderthals due to faster maturation rates [31] ). However, due to this very early maturation ontogenetic changes of adjacent and surrounding facial structures, growing much longer than the cribriform plate [32] , are very unlikely to influence cribriform morphology by craniofacial integration. Moreover, the fact that large-faced Neanderthals showed smaller cribriform plates supports an interpretation in terms of neurological factors rather than by craniofacial integration. Furthermore, its specific increase in H. sapiens implies a unique evolutionary condition of a large cribriform plate atop a nasal cavity within an extremely reduced face [2] , [27] . After all, nasal cavity and facial sizes are more related to respiration and mastication than to olfaction [32] . Cribriform expansion also explains Lieberman et al . 's [2] suggestion that modern humans have increased relative length of the anterior cranial base at the midline floor, because that length is composed of both, the cribriform plate and the pre-sphenoid, the latter of which is not distinctive between archaic and modern humans [13] ( Supplementary Discussion ). Other basicranial structures mature morphologically later in ontogeny and their interactions with other craniofacial elements are more complex. For example, the midline basicranium attains adult morphology around 6 years of age in modern humans [32] , [33] . The primate midline cranial base is not only determined by the morphology of the brain [34] but also by intrinsic factors of its endocranial precursors [9] and by facial size [35] . Although in primates large brains are associated with more flexed cranial bases, larger faces are associated with less basicranial flexion [35] , which explains why large-brained and large-faced Neanderthals have less flexed cranial bases than equally large-brained, but small-faced modern humans [35] . The lateral cranial base (ACF, MCF) matures later in ontogeny than midline structures, although still about 4 years earlier than the face [32] . This dissociation offers potential for morphological interaction of the endocranial base with the brain and the neurocranium on its top, and the face below [30] , [32] . However, the volume of the MCF scales isometrically with that of the temporal lobes [27] , indicating developmental integration, which corresponds with their common embryological origin (ecto- and endomeninx) [9] , [10] , and strongly supports neurological interpretations of MCF morphology. The association between the frontal lobes and the ACF is less well studied. Bookstein et al . [36] suggested that the shape of the frontal lobes in the midline has remained unchanged since the Middle Pleistocene, despite significant evolutionary modifications of facial morphology. Furthermore Stedman et al . 's [37] data show that genetic factors of masticatory apparatus and facial development were not likely relevant for frontal lobe evolution after early Homo . More research is needed on the integration between the frontal lobes, the ACF, the cribriform plate and facial morphology ( Supplementary Discussion ). At a functional level, variation of olfactory bulbs size is crucially related to olfactory capacity and performance, which has been observed across [38] , [39] , [40] , [41] and within [42] species. Olfactory bulb size differences are also the morphofunctional basis of traditional distinctions between macrosmatic and microsmatic mammals regarding subsistence strategies and other features of animal behaviour [38] , [39] , [40] , [41] . In addition, within humans, the capacity of odour threshold detection and odour identification is correlated positively with olfactory bulb size, which is driven by variation in the number of nerve cells [41] , [42] . The number of cells relates more to olfactory function than overall volume of the olfactory bulbs, which is why Smith (ref. 41 ), personal communication) suggested that in closely related organisms with roughly comparable size and similar overall cribriform plate morphology, or in intraspecific comparisons, correction for scaling 'needlessly complicates' functional interpretations. Therefore, the ca. 12% larger cribriform plates and associated larger olfactory bulbs in modern humans may be suggestive of improved olfactory function [11] , [42] , [43] , although caution is warranted because of the small Neanderthal sample. Further comparative anatomical study has reported that increase of olfactory bulb volume relative to brain size correlates with volume increase in a number of other functionally related limbic structures [30] , located at basal parts of the brain including the temporal lobes (for example, hippocampus, amygdala). Recent brain mapping research using functional magnetic resonance imaging has shown links between neocortical counterparts of ACF and olfactory and gustatory function [23] . Olfactory and gustatory function, due to its rewarding characteristics and links to memory, was also suggested to participate in an effective and flexible human learning system [23] , [43] . Moreover, positron emission tomography data of regional cerebral blood flow confirmed involvement of the orbitofrontal cortex in processing emotionally valenced olfactory stimuli and decision making [22] , [44] . However, the volume of the human frontal lobes does not apparently differ from that of other hominoids, taking allometric scaling into account [14] , [15] , although some evidence starts to emerge that 'shape (and not volume)' is relevant to brain function at specific structures [45] . Whether shape differences at the basal frontal lobes of large-brained humans ( Figs 4 and 5 ) reflect different functional features or are consequences of craniofacial integration must remain speculative and requires further investigation ( Supplementary Discussion ). Currently, developmental and evolutionary interactions between the frontal lobe base at the ACF and the cribriform plate may be the safest assumption. However, the coincident evolutionary changes of structures comprising olfactory neuro-circuitry could be a novel feature in the evolution of H. sapiens , and, if confirmed, may have influenced some features of human behaviour. The olfactory neurological circuitry is highly integrated in cerebral, behavioural and immunological functions [44] , [46] . Following the initial sensory process, axons from thousands of cells expressing odour receptors in the mucosa of the nasal cavity converge via the cribriform plate in the olfactory bulb [38] , [39] , [40] , [41] . From there, olfactory signals are transmitted to the olfactory cortex (rhinal, pyriform cortex, medioventral to temporal lobe poles) and become relayed, on the one hand to higher cortical regions, where conscious thought processes are handled, and on the other hand to the limbic system, where emotional context is generated [38] , [43] , [44] . Olfactory information thus projects to regions critical for mating, emotions, and fear (amygdala) as well as for motivation, high-level cognitive and emotional processes (orbital prefrontal cortex). It, thus, serves a role in central nervous system function above and beyond smell [46] , [47] . In that respect, olfaction differs from other sensory modalities. Odour immediately triggers strong emotional evocations and provokes higher memory retention ('Marcel Proust Phenomenon') due to anatomical overlap of structures involved in memory process and olfaction pathways [43] . Such associations with cognitive processes have been termed by Savic [44] 'higher olfactory functions'. Smell, and linked higher olfactory functions, can thus be involved in modulating many different aspects of human behavior [43] , [44] , [46] , [47] . It has been reported that people who are congenitally deaf or blind have intact reproductive–social capacities, whereas individuals with congenital anosmia usually do not [43] . Moreover, olfaction has been linked to the immunological system [46] . It is speculated that odour might be an important factor of attractiveness, that is, a mate selection criterion in human females, possibly selected for improving immunological fitness of the offspring, for example, in the case of the major histocompatibility complex [46] , [48] . Other recent research suggests that humans are also able to detect the 'scent of fear' [49] , potentially important in human social interaction. Bruner et al . [6] suggested that Neanderthals possess—in general—an encephalized (enlarged) version of a primitive Homo brain by being at the endpoint of an archaic allometric trajectory, significantly different from the modern human brain scaling trajectory [6] . On the other hand, a more localized study revealed also the width of the Neanderthal frontal lobes to be non-allometrically increased [12] . Our results may fit with these observations. Figure 1 , indicating roughly parallel distributions of archaic and modern human scatters, likely reflects some of these general differences, and resembles plots of Bruner et al . [6] Different scaling also seems consistent with recent studies of endocranial development showing that Neanderthal brains grew differently early in ontogeny, and probably prenatally, when compared with modern humans [7] . Evolutionary differences comprise the entire craniofacial system [7] , [50] , [51] . Detailed basicranial comparisons between Neanderthals and modern humans have been missing so far and our study fills that gap. On the basis of previously mentioned investigations, and also the findings of this study, it is hypothesized that their smaller olfactory bulbs ( Fig. 5g,h ) relate to differences in scaling patterns between Neanderthals and modern humans [6] , [7] . Our findings support previous hypotheses [6] , [7] that modern humans show a different evolutionary trajectory because of the remaining significant shape differences between Neanderthals and H. sapiens after allometric size adjustment ( Fig. 5 , Table 2 ). Different evolutionary patterns likewise emerge from comparative genetic analyses, which—among other aspects—have shown evidence for positive selection of genes related to cognitive development, that occurred after the split of H. sapiens and Neanderthals [5] . The same applies to roughly 4% of the 78 amino-acid configurations, which—ancestral in Neanderthals—are directly related to the olfactory system [5] . Differences in the configuration of the olfactory sensory apparatus, and its previously discussed involvement into higher olfactory functions in social, and cognitive (memory) aspects [43] , [44] , [47] could be part of this evolutionary process. Care should be taken when interpreting our findings by invoking evolutionary mechanisms that might have favored a better capacity of smell in modern humans compared with Neanderthals in a way analogous to macrosmatic and microsmatic mammals [39] , [40] , [41] . Rather, olfaction-related circuitry, as part of a wider integrated functional and structural neuronal network, may have been favored in the evolution of H. sapiens in a social context. However, olfaction, and its contribution to gustation with its links to reward (pleasure) [23] and memory, could also be of evolutionary relevance, but at a secondary level [27] regarding the manipulation of food [23] , [52] . Although it has been speculated that early modern humans may have fed on a wider array than Neanderthals [53] , the role that olfaction, gustation or memory and reward might have had in this context must remain open to speculation. Lieberman [27] suggested that the effect of higher basicranial flexion, approximating pharynx and olfactory epithelium, has enhanced the retronasal contribution of smell to taste [52] . Evolutionary changes at the cribriform plate and the associated olfactory bulbs [11] , [42] and other endocranial parts we report here can implicate changes to the olfactory system that appear unique to modern humans. It is clear, however, that cognitive functions are incommensurable even with the most sophisticated measurement of brain impressions in endocranial casts. Therefore, palaeoneurological interpretation of evolutionary variations in cerebral surface such as reflected in the basal endocranium in functional terms remains a challenge [3] , [6] , [7] , [8] , [12] . Although different regions of the prefrontal cortex (frontal lobes) have been associated with higher integrative and social functions, (for example, decision making) [12] , [20] , [21] , [22] , [23] , [24] , regions of the temporal lobes are traditionally related to visual memory, language and to theory of mind [24] , [54] , [55] . All of them are compatible with higher olfactory functions [44] . Our study provides a much needed palaeontological basis [52] , which draws neuroscientific attention to further investigation of these structures. Palaeontological data can indicate when during human evolution such structural changes and putative sets of associated systems have occurred. We show that specimens attributable to early H. sapiens are within the range of modern configurations of the endocranial base of the brain, thus suggesting a first appearance at least approximately 130 kyr ago (for example, Singa) [56] . We conclude that the evolution of the base of the brain in highly encephalized human species produced significant differences in early Homo–H. neanderthalensis evolutionary trajectory compared with those observed in early Homo– H. sapiens , at basal frontal and temporal lobes, the details of which have never shown before. And surprisingly, although both human species showed increase at the cribriform plates and olfactory bulbs, the spatial position of these structures within the brain differed significantly. Increased cribriform plates suggests larger olfactory bulbs [11] , [38] , [39] , [40] , [41] in modern humans. This does not only fit with the relative enlargement of midline anterior cranial floor suggested previously [2] , [27] but also elucidates why, morphologically and when, chronologically this happened in human evolution. One likely framework for the palaeoneurological interpretation of these data points to higher olfactory functions ( sensu Savic [44] ) in H. sapiens , because all structures in this evolutionary process share intimate relations to this sensory modality. 'Higher olfactory' functions [44] relate odour reception with socially relevant cognitive processes, for example, subliminally smell-mediated modulation of human-specific behavior [43] , [47] . Other possible factors may relate to the immunological system [46] , fear [49] , kinship or group recognition [4] , [43] , [47] ) or food manipulation [27] , [52] , [53] and could be among the implications of these new findings on the evolution of the basal areas of the human brain. Landmarks and digitizing procedure A set of 158 3-D landmarks and semilandmarks was digitized by hand on the endocranial surface of the cranial base on 3-D reconstructions of computed tomography scans. These landmarks define both structures traditionally measured at the cranial base as well as specifically endocranial 3-D surface morphology of the base of the frontal and temporal lobes ( Supplementary Table S1 ; Supplementary Fig. S1 ). Computed tomographic scans of 30 common chimpanzees ( P. troglodytes verus ) and 75 adult recent humans representing geographic variation from Africa, Asia and Europe, and 14 fossil Pleistocene humans ( Table 1 ) were reconstructed and computer models of their 3-D endocranial surfaces were generated in Amira 4.1 software (Mercury Inc.). Shape data were recorded by landmarks on these 3-D endocranial surfaces. Landmark digitizing error was small, as reported elsewhere [16] . The fossils were also digitized by hand in Amira 4.1. Missing data due to taphonomic factors were carefully estimated following standard estimation methods available for semilandmark data [57] . Missing data estimation was performed conservatively using the modern human template ( Supplementary Fig. S1 ) for TPS estimation by Morpheus et al . ( www.morphometrics.org ). The reconstructed landmarks were then projected onto 3-D surface models of reconstructed fossils and edited further by hand in ViewBox4 ( www.dhal.com ) and Edgewarp software ( http://brainmap.stat.washington.edu/edgewarp ). Thin-plate splines were used iteratively for minimizing the bending energy between the modern human average and the fossil during the sliding, re-sliding and re-projection procedure [17] , [57] . Before statistical analyses landmark data were symmetrized [17] , [57] , because in some cases (KNM-ER 3733, KNM-ER 3883) an acceptable correction to shear taphonomic deformation was obtained [57] ( Fig. 6 ), and because studying asymmetry (petalia) was not an aim of the study. 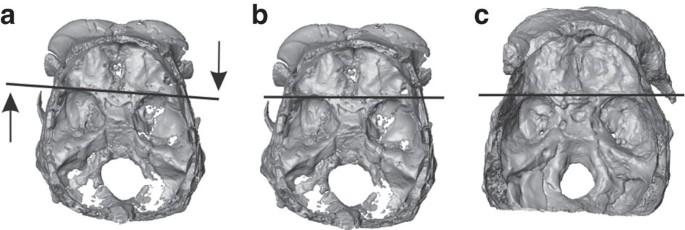Figure 6: Virtual reconstruction of taphonomic deformations in earlyHomosample. (a) Original endocranial surface of the base of the brain of KNM-ER 3733 (taphonomic shear, indicated by arrows, causes anatomical distortion shown by tilted line; (b) reconstructed surface of the same fossil (note the horizontal position of the previously rotated line); (c) endocranial view of KNM-ER 3883 showing only minor deformations at the endocranial base of the brain. Figure 6: Virtual reconstruction of taphonomic deformations in early Homo sample. ( a ) Original endocranial surface of the base of the brain of KNM-ER 3733 (taphonomic shear, indicated by arrows, causes anatomical distortion shown by tilted line; ( b ) reconstructed surface of the same fossil (note the horizontal position of the previously rotated line); ( c ) endocranial view of KNM-ER 3883 showing only minor deformations at the endocranial base of the brain. Full size image Statistical analyses Principal components analysis in form space, multivariate regression analyses and mean shape comparisons were performed using routines programmed by Philipp Gunz and Philipp Mitteroecker [17] , MorphoJ ( www.flywings.org.uk ) and the EVAN-toolbox ( www.evan-society.org ). During 10,000 permutations, group sizes were kept constant but group membership was re-sampled. The test assessed the statistical significance of the observed mean Procrustes distance between species means, comparing how often mean distances were obtained equal to or greater than the observed ones due to random group membership. Wald–Wolfowitz runs [58] test was performed using Statistica 8.0 (StatSoft Inc.) to test the null hypothesis that cribriform length measurements were drawn from the same sample. It expects the data to be arranged in the same way as the t -test does for independent samples, but does not make any assumption on normality. It is, thus, a useful test when very small sample sizes preclude using traditional parametric statistics (such as Student's t -test). In addition, in small samples, z -adjustments have been recommended [58] . Visualizations and TPS Finally, the EVAN toolbox was used for calculation and visualization of specifically located TPS in mean shape differences. These splines are registration-independent interpolations between two landmark configurations, and most informative in their closest vicinity [16] , [17] , [57] . Splines were used to illustrate hypothesis-related features of shape differences between the species means. Several TPS-grids were calculated according to the anatomical hypothesis. The ACF TPS-grid was defined by endocranial regions close to landmarks 10, 20, 48, 65, 108 ( Supplementary Table S1; Supplementary Fig. S1 ). The MCF TPS-grid was positioned close to lms 16, 26, the anterior poles of the temporal lobes within the greater sphenoid wings (landmarks 11, 16, 21 and 26) ( Supplementary Table S1; Supplementary Fig. S1 ) [26] . A vertical TPS-grid was calculated close to landmarks 16 and 26 and the lesser sphenoid wings, to indicate the antero–posterior variation of the midline base due to evolutionary changes at the cribriform plate relative to the lateral endocranial antero–posterior shifts. Cribriform shape was further visualized by local white-coloured TPS-grid through its delimiting landmarks 2, 3, 4, 18 and 19 ( Supplementary Table S1; Supplementary Fig. S1 ). How to cite this article: Bastir, M. et al . Evolution of the base of the brain in highly encephalised human species. Nat. Commun. 2:588 doi: 10.1038/ncomms1593 (2011).